Single-molecule force spectroscopy reveals force-enhanced binding of calcium ions by gelsolin Force is increasingly recognized as an important element in controlling biological processes. Forces can deform native protein conformations leading to protein-specific effects. Protein–protein binding affinities may be decreased, or novel protein–protein interaction sites may be revealed, on mechanically stressing one or more components. Here we demonstrate that the calcium-binding affinity of the sixth domain of the actin-binding protein gelsolin (G6) can be enhanced by mechanical force. Our kinetic model suggests that the calcium-binding affinity of G6 increases exponentially with force, up to the point of G6 unfolding. This implies that gelsolin may be activated at lower calcium ion levels when subjected to tensile forces. The demonstration that cation–protein binding affinities can be force-dependent provides a new understanding of the complex behaviour of cation-regulated proteins in stressful cellular environments, such as those found in the cytoskeleton-rich leading edge and at cell adhesions. Gelsolin is an actin-binding protein that regulates the architecture of the actin cytoskeleton by severing, capping and uncapping actin filaments [1] , [2] . Through controlling actin organization, gelsolin influences cellular processes, such as cell motility, apoptosis, phagocytosis and platelet activation [3] . To perform these functions, gelsolin needs to cycle between activated and inactivated states, which are largely regulated by calcium ion concentrations ([Ca 2+ ]). Under physiological conditions, half-maximal activity of gelsolin requires a calcium concentration of ~10 μM, but this can be significantly decreased by lowering the pH or through tyrosine phosphorylation [4] , [5] . The sixth domain of gelsolin (G6) serves as the gatekeeper of the globular inactive protein. Upon calcium binding, the kinked central helix of G6 is straightened ( Fig. 1a,b ), which is proposed to trigger the separation of the C-terminal helix of G6 from the second domain (G2), transforming the inactive globular form of gelsolin into an extended pearl-necklace-like active form [6] , [7] , [8] . Molecular dynamics simulations on G6 and structural comparisons with its homologous domain from villin, V6, indicate that the calcium-free structure of the sixth domain is held in a strained conformation within the intact protein due to interactions with the sequences outside G6 (ref. 9 ). During the activation of gelsolin, domains G3 and G6 undergo large rotations and translations of >40 Å with respect to the neighbouring domains. Such conformational changes may lead to tensile forces being generated between the domains. 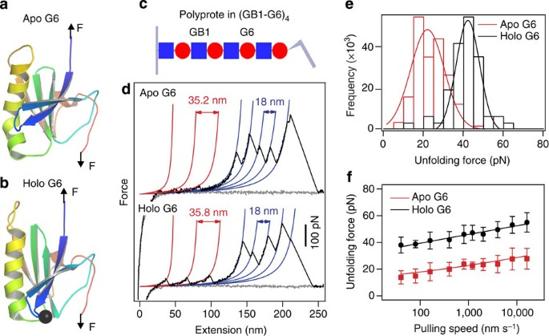Figure 1: Mechanical properties of G6 probed by single-molecule AFM. The structure of G6 in the absence of Ca2+(PDB ID: 3FFN) (a) and in the presence of Ca2+(shown as black sphere), (PDB ID: 1P8X) (b). Upon Ca2+binding, the central long helix is straightened. The schematic representations are shown in rainbow colours from blue (N termini) to red (C termini). The C-terminal latch sequence is not shown because it becomes unstructured in holo G6 and was not evident in the crystal structures of gelsolin-actin complexes (Supplementary Fig. 1). However, the C-terminal helix sequence was included in the polyprotein (GB1–G6)4for single-molecule AFM experiments. The arrows indicate the direction of applied force is from the N to C terminus of G6. (c) A schematic of the hetero-polyprotein (GB1–G6)4used for single-molecule force spectroscopy experiments. Red circles and blue squares represent G6 and GB1 domains, respectively. (d) Typical set of approaching (grey line) and retraction traces for mechanical unfolding of calcium-free apo or calcium-bound holo forms of (GB1–G6)4at a pulling speed of 400 nm s−1. WLC fitting of consecutive unfolding events (red and blue lines) identifies that all saw-tooth-like peaks result from the unfolding of G6 and GB1 domains with contour length increments of 35 nm and 18 nm, respectively. The unfolding force for G6 increases from ~20 to ~40 pN upon saturation with Ca2+(at ~50 μM) while the unfolding force for GB1 remains the same. (e) Unfolding force histograms of apo and holo G6. (f) Pulling speed dependency of apo and holo G6. The unfolding force increases with increasing pulling speed. Error bars represent standard deviations. The experimental data can be numerically fitted using a two-state unfolding model (solid lines). The unfolding rate constant at zero force (k0) and the unfolding distance (Δxu) are 0.09 s−1and 1.73 nm for apo G6, and 5.0 × 10−5s−1and 1.60 nm for holo G6, respectively. Figure 1: Mechanical properties of G6 probed by single-molecule AFM. The structure of G6 in the absence of Ca 2+ (PDB ID: 3FFN) ( a ) and in the presence of Ca 2+ (shown as black sphere), (PDB ID: 1P8X) ( b ). Upon Ca 2+ binding, the central long helix is straightened. The schematic representations are shown in rainbow colours from blue (N termini) to red (C termini). The C-terminal latch sequence is not shown because it becomes unstructured in holo G6 and was not evident in the crystal structures of gelsolin-actin complexes ( Supplementary Fig. 1 ). However, the C-terminal helix sequence was included in the polyprotein (GB1–G6) 4 for single-molecule AFM experiments. The arrows indicate the direction of applied force is from the N to C terminus of G6. ( c ) A schematic of the hetero-polyprotein (GB1–G6) 4 used for single-molecule force spectroscopy experiments. Red circles and blue squares represent G6 and GB1 domains, respectively. ( d ) Typical set of approaching (grey line) and retraction traces for mechanical unfolding of calcium-free apo or calcium-bound holo forms of (GB1–G6) 4 at a pulling speed of 400 nm s −1 . WLC fitting of consecutive unfolding events (red and blue lines) identifies that all saw-tooth-like peaks result from the unfolding of G6 and GB1 domains with contour length increments of 35 nm and 18 nm, respectively. The unfolding force for G6 increases from ~20 to ~40 pN upon saturation with Ca 2+ (at ~50 μM) while the unfolding force for GB1 remains the same. ( e ) Unfolding force histograms of apo and holo G6. ( f ) Pulling speed dependency of apo and holo G6. The unfolding force increases with increasing pulling speed. Error bars represent standard deviations. The experimental data can be numerically fitted using a two-state unfolding model (solid lines). The unfolding rate constant at zero force (k 0 ) and the unfolding distance ( Δx u ) are 0.09 s −1 and 1.73 nm for apo G6, and 5.0 × 10 −5 s −1 and 1.60 nm for holo G6, respectively. Full size image Although it has been predicted that force can alter the native structure of biomolecules, and consequently their affinities for ligands, experimentally verifying such predictions remains challenging [10] , [11] , [12] , [13] , [14] . In particular, it was difficult to quantitatively measure the binding affinities of ligands in the presence of different forces. With the development of single-molecule force spectroscopy techniques, it is now possible to apply forces to individual biomolecules and study their folding/unfolding and structural dynamics [15] , [16] , [17] , [18] , [19] . Recently, we and others have established a force spectroscopy based binding assay to directly measure the equilibrium dissociation constants ( K d ) of ligands to proteins at the single-molecule level, based on different mechanical stabilities of the ligand-bound and ligand-free forms of proteins [20] , [21] . This method was established for a slow-exchange ligand system, where the binding and dissociation of ligands from proteins during the force spectroscopy experiments can be neglected. Here we extended this method to address whether force can regulate calcium binding of G6 and thus influence function of gelsolin. We find that the binding of calcium ions to G6 is a fast equilibrium. By considering the exchange rate between calcium-free and calcium-bound forms, we are able to quantify the K d of the interaction between calcium ions and G6. We determine that the dissociation constant of this interaction is force-dependent, and moreover and somewhat counter-intuitively, our model suggests that the applied tensile force increases, rather than decreases, the binding affinity. Our results imply that G6 can be activated at lower calcium concentrations when subjected to tensile forces from neighbouring domains during conformational changes. Inter-domain tensions will be an inbuilt feature of multiple-domain proteins. Thus, this may serve as a general mechanism for cooperativity and communication between domains. Mechanical stability of calcium-free and calcium-bound G6 To study the unfolding of G6 ( Supplementary Fig. 1 ) using atomic force microscopy (AFM) based single-molecule force spectroscopy, we engineered a soluble, folded polyprotein (GB1–G6) 4 ( Fig. 1c and Supplementary Fig. 2 ), in which G6 is spliced alternatively with the well-characterized protein domain GB1 (refs 22 , 23 ). The mechanical unfolding features of GB1 serve as a fingerprint to identify the mechanical unfolding signal of G6 (ref. 24 ). GB1 neither shows any measurable interactions with G6 nor affects the calcium-binding affinity of G6 ( Supplementary Fig. 3 ). GB1 also does not change the thermal stability of G6 ( Supplementary Fig. 4 ). The mechanical stability of GB1 remains the same in the presence of calcium ions ( Supplementary Fig. 5 ). Taken together, these results demonstrate GB1 to be an ideal fingerprint protein for the study of the calcium binding of G6 in single-molecule AFM experiments. (GB1–G6) 4 was stretched by physical adsorption between a cantilever tip and a glass surface. Due to such an uncontrolled attachment strategy, the number of protein domains being unfolded varies in different unfolding traces, as has been well-documented [25] . The force-extension curves of (GB1–G6) 4 are characterized by saw-tooth-like unfolding patterns ( Fig. 1d ) in which lower-force unfolding peaks are followed by higher-force unfolding peaks of ~150 pN and a contour length increment ( ΔL c) of ~18 nm that correspond to the unfolding of GB1 in the polyprotein [22] , [23] , [24] . Since G6 alternates with GB1 within the hybrid polyprotein, the lower-force peaks preceding GB1 unfolding events result from the mechanical unfolding of G6. Fitting the unfolding events of G6 using the worm-like chain (WLC) model for polymer elasticity yields a ΔL c of 35.2±3.2 nm (mean±s.d., n =150). The enlarged figure displaying the WLC fittings to the unfolding events of G6 is shown in Supplementary Fig. 6 . Since G6 comprises of 116 amino acids (640–755 of gelsolin) and the distance between the N and C termini of a folded G6 domain in its apo form is 3.5 nm, stretching a G6 domain from the folded state to the unfolded state should give rise to a contour length increment of 38.8–42.9 nm (0.365–0.4 nm were chosen for the contour length per amino acid; 0.365–0.4 nm/aa × 116 aa–3.5 nm=38.8–42.9 nm). The difference between our experimentally measured and the calculated values may come from the unfolding of the C-terminal extension to G6 (residues 737–755, Supplementary Fig. 1 ). The unfolding force for calcium-free G6 is 23.9±6.1 pN (mean±s.d., n =150), indicating the low mechanical stability of G6. However, at a saturating calcium concentration of 50 μM, the unfolding force increases dramatically to 41.0±6.1 pN (mean±s.d., n =171), indicating that the mechanical stability of G6 is increased by calcium binding. The unfolding force distributions for calcium-free and calcium-bound G6 are summarized in Fig. 1e . To make sure such an increase in the unfolding force for G6 was not simply due to a change in ionic strength of the solution on addition of calcium ions, we performed single-molecule AFM experiments on (GB1–G6) 4 in the presence of 5 mM magnesium ions ( Supplementary Fig. 7 ). The unfolding forces determined for G6 and GB1 are both unaffected by the presence of magnesium ions, suggesting that the observed increase in mechanical stability of G6 is not due to non-specific binding at elevated ionic strength. In the presence of saturating levels of calcium ions, the contour length increment of G6 remains unchanged at 35.4±3.0 nm (mean±s.d., n =171). Therefore, the C-terminal extension to G6 still unfolds before the unfolding of the rest of the G6 domain. To further illustrate this, we measured the contour length increment of G6 and GB1 at various concentrations of calcium ions ( Supplementary Fig. 8 ). The contour length increment of G6 remains unchanged, even at a [Ca 2+ ] of 5 mM. To obtain the kinetic parameters underlying the free energy landscape of the unfolding of calcium-free and calcium-bound G6, we measured the average unfolding force at different pulling speeds. Consistent with most other proteins that have been studied using single-molecule AFM, the unfolding force for both forms of G6 increase logarithmically with respect to pulling speed ( Fig. 1f ). This pulling speed dependency can be adequately reproduced by numerical fitting using either a simple two-state unfolding model [26] , [27] or a Monte Carlo simulation [28] ( Supplementary Material , Supplementary Fig. 9 ). The spontaneous unfolding rates for calcium-free and calcium-bound G6 ( k ua0 and k uh0 ) are 0.09 s −1 and 5.0 × 10 −5 s −1 , respectively, and the unfolding distances for calcium-free (apo) and calcium-bound (holo) G6 ( Δx ua and Δx uh ) are 1.73 nm and 1.60 nm, respectively. Unimodal unfolding force distributions for G6 at intermediate [Ca 2+ ] To obtain the binding isotherm describing the interaction between calcium and G6, we studied the unfolding force distribution for G6 at intermediate [Ca 2+ ]. For slow-exchange ligands, the dissociation and association of ligands can be neglected in force spectroscopy experiments. The apo and holo forms of a protein can coexist at intermediate ligand concentrations. However, the unfolding force for G6 is in sharp contrast with those of slow-exchange ligand binding proteins at non-saturating [Ca 2+ ]. As shown in Fig. 2a , instead of observing two populations of unfolding forces of ~20 pN and ~40 pN corresponding to calcium-free and calcium-bound forms, respectively, we found a gradual shift of the unfolding force for G6 along with an increase of [Ca 2+ ], from 23.9±6.1 pN in the absence of calcium to 34.2±7.0 pN at 5 μM, and to 38.1±7.5 pN at 25 μM. Further increase of [Ca 2+ ] has little effect on the unfolding force for G6, indicating that the calcium-binding site is saturated at ~25 μM. To more precisely describe the variation of unfolding force at different calcium concentrations, we summarize the unfolding force histograms for G6 from many single-molecule trajectories ( Fig. 2b ). Clearly, these histograms show unimodal distributions without a clear distinction between the calcium-free and calcium-bound forms. Moreover, the widths of the distributions are ~10 pN at each [Ca 2+ ] studied. This suggests that the unimodal unfolding force distributions are not the simple sum of unfolding events of calcium-free and calcium-bound forms. Since G6 can only adopt calcium-free and calcium-bound structures, it is intriguing to observe such an ‘averaged’ conformation of G6 that shows intermediate mechanical stabilities. Similar gradual increase of mechanical unfolding forces upon metal ion binding has also been observed for calmodulin and this was hypothesized to arise from the fast equilibrium of the apo and holo conformations [29] . There might be other explanations for the observed unimodal distribution of forces at intermediate concentrations. For example, G6 may undergo continuous structural changes upon the increasing calcium concentrations; however, such a model is not supported by structural biology which has identified a single Ca 2+ -binding site in G6 ( Fig. 1b ). Nonetheless, such a unimodal distribution of unfolding forces at intermediate calcium concentrations makes it impossible to calculate directly the contributions of the bound and unbound forms of G6 from force-extension traces. A kinetic model that considers the interconversion rates between calcium-free and calcium-bound forms is required to obtain the dissociation constant. 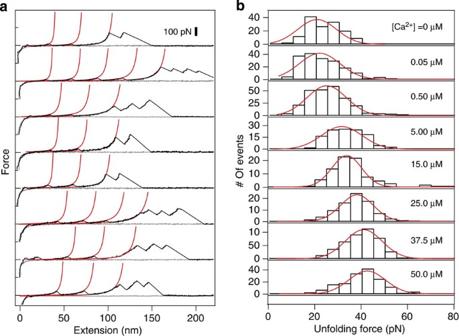Figure 2: Mechanical unfolding of G6 at different [Ca2+]. (a) Representative force-extension profiles for unfolding of (GB1–G6)4in the presence of various [Ca2+] at a pulling speed of 400 nm s−1. The [Ca2+] at which the traces were measured are shown on the same row inb. Red lines correspond to the WLC fitting to the G6 unfolding events. (b) The unfolding forces histograms at different [Ca2+]. The solid lines are Gaussian fittings of these data. The unfolding forces of G6 show unimodal distributions at all Ca2+concentrations and the widths of the distributions remain constant. This indicates that the calcium-free and calcium-bound conformations are in fast equilibrium upon stretching. Figure 2: Mechanical unfolding of G6 at different [Ca 2+ ]. ( a ) Representative force-extension profiles for unfolding of (GB1–G6) 4 in the presence of various [Ca 2+ ] at a pulling speed of 400 nm s −1 . The [Ca 2+ ] at which the traces were measured are shown on the same row in b . Red lines correspond to the WLC fitting to the G6 unfolding events. ( b ) The unfolding forces histograms at different [Ca 2+ ]. The solid lines are Gaussian fittings of these data. The unfolding forces of G6 show unimodal distributions at all Ca 2+ concentrations and the widths of the distributions remain constant. This indicates that the calcium-free and calcium-bound conformations are in fast equilibrium upon stretching. Full size image A force-independent binding model In this trial, and ultimately unsuccessful, model, we consider the effect of a dynamic equilibrium between the calcium-free and calcium-bound forms of G6 on the unfolding force for G6. As shown in Fig. 3a , there are two different types of kinetics involved: the calcium-dependent interconversion kinetics between calcium-free and calcium-bound forms of G6 and the force-dependent unfolding kinetics of the calcium-free and calcium-bound forms. Since the interconversion between calcium-free and calcium-bound forms is force independent, we term this model as a ‘force-independent binding model’. We define the conversion rate from calcium-free to calcium-bound as k on and the reverse conversion rate as k off . 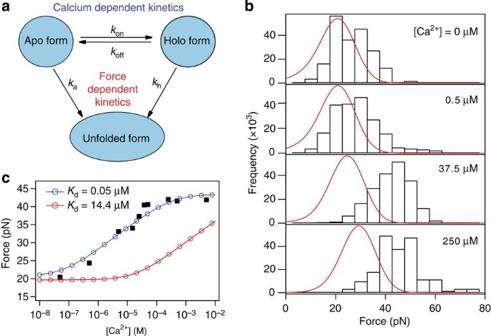Figure 3: A force-independent binding model. (a) The kinetic model that considers rapid dynamics between the calcium-free apo and the calcium-bound holo conformations. The unfolding of both the apo and holo forms are force-dependent processes and the interconversion between the apo and holo forms depends on the calcium concentration and is force independent. (b) This kinetic model fails to reproduce the unfolding force histograms at various calcium concentrations. Black bars correspond to the experimentally obtained unfolding force histograms and red lines correspond to the numeric fitting results using the kinetic model depicted inaTheχ2for the fittings to the histograms from top to bottom are 0.093, 0.096, 0.308 and 0.290, respectively. (c) This kinetic model cannot describe the unfolding forces of G6 at different calcium concentrations. Red circles correspond to the numerically calculated data using aKdof 14.4 μM, as determined from ITC measurements. Blue circles correspond to the numerically calculated data using aKdof 0.05 μM that best ‘fits’ the experimental data. However, the slope of the unfolding force versus [Ca2+] relationship cannot be fully reproduced. Theχ2for numerically calculated data usingKds of 14.4 and 0.05 μM are 14.0 and 0.33, respectively. Therefore, Figure 3: A force-independent binding model. ( a ) The kinetic model that considers rapid dynamics between the calcium-free apo and the calcium-bound holo conformations. The unfolding of both the apo and holo forms are force-dependent processes and the interconversion between the apo and holo forms depends on the calcium concentration and is force independent. ( b ) This kinetic model fails to reproduce the unfolding force histograms at various calcium concentrations. Black bars correspond to the experimentally obtained unfolding force histograms and red lines correspond to the numeric fitting results using the kinetic model depicted in a The χ 2 for the fittings to the histograms from top to bottom are 0.093, 0.096, 0.308 and 0.290, respectively. ( c ) This kinetic model cannot describe the unfolding forces of G6 at different calcium concentrations. Red circles correspond to the numerically calculated data using a K d of 14.4 μM, as determined from ITC measurements. Blue circles correspond to the numerically calculated data using a K d of 0.05 μM that best ‘fits’ the experimental data. However, the slope of the unfolding force versus [Ca 2+ ] relationship cannot be fully reproduced. The χ 2 for numerically calculated data using K d s of 14.4 and 0.05 μM are 14.0 and 0.33, respectively. Full size image where, k m is the cation binding rate; [Ca 2+ ] is the calcium ion concentration; and K d is the equilibrium dissociation constant, which was measured using isothermal titration calorimetry (ITC) ( Supplementary Fig. 3 ). The unfolding rates for the apo calcium-free form ( k ua ) and the holo calcium-bound form ( k uh ) can be estimated using the Bell–Evans equation as follows [30] , [31] : wHere k ua0 , k uh0 , Δx ua and Δx uh are as defined as above; β =1/ k B T ( k B is the Boltzmann constant; and T is the absolute temperature). F ( t ) is the applied force at time t , which can be calculated using a WLC model [32] . where, v is the pulling speed; p is the persistence length; L c is the contour length; and β is as defined above. Using numerical fitting, we estimate the effect of k on and k off on the unfolding forces of G6 at the intermediate [Ca 2+ ] of 25 μM ( Supplementary Fig. 10 ). Although the interconversion kinetics between the calcium-free and calcium-bound states is not directly associated with the force-dependent unfolding rates, it significantly affects the unfolding force for G6 through a kinetic network depicted in Fig. 3a . At a cation dissociation rate, k off , <10 s −1 , the unfolding forces for the calcium-free and calcium-bound G6 are well-separated in the unfolding force histograms and show a bimodal distribution ( Supplementary Fig. 10 ). However, when the cation dissociation rate is >10 s −1 and <400 s −1 , the unfolding forces for the calcium-free and calcium-bound G6 gradually shift towards each other and merge into a single broad distribution. Further increase in the cation binding rate leads to the complete degeneration of the unfolding force histogram into a combined, unimodal distribution, characterized by a width of the distribution similar to those calculated for the individual calcium-free and calcium-bound forms. Based on this simulation, it is clear that the calcium-binding rate to G6 should be more than 1.7 × 10 3 s −1 to warrant a single unimodal unfolding force distribution for G6 at the intermediate calcium concentration ( k off >1,000 s −1 ). However, while this kinetic model can adequately reproduce the unimodal distribution of unfolding forces at the intermediate [Ca 2+ ], it fails to match the average unfolding forces ( Supplementary Fig. 10 and Fig. 3b ). Such a deviation is not unique to a particular data set at a given [Ca 2+ ] but a common feature for the unfolding force distributions for G6 across a range of calcium concentrations ( Fig. 3b ). Moreover, the experimentally measured forces vary with the [Ca 2+ ], a behaviour that is not predicted by the simulated unfolding forces ( Fig. 3b ). The average unfolding forces from both experimental and numerical fittings at different calcium concentrations are summarized in Fig. 3c . Clearly, using the K d obtained from the ITC measurements (14.4 μM), the simulated unfolding forces are much lower than those from the experiments. In AFM experiments, proteins are tethered on the surface and the cantilever tip. Surface tethering could possibly affect calcium binding due to geometric restrictions, leading to a slight increase in K d ; however the polyprotein approach used here should overcome any such effect. To match the unfolding forces, we need to assume a K d of 0.05 μM, which is ~280 fold smaller than that obtained from the ITC measurement and is lower than the measured K d for any known gelsolin domain determined using a variety of experimental methods (0.1–50 μM) [4] , [5] , [33] , [34] , [35] , [36] , [37] . Moreover, even with such an artificially low ‘assumed’ K d , the slope of the change of unfolding force with respect to the [Ca 2+ ] cannot be fully reproduced in the simulation. Therefore, a more accurate kinetic model is required to understand the dynamics of G6 under force. A force-dependent binding model In the second kinetic model, we consider that the unfolding kinetics of the calcium-free and calcium-bound forms, and their interconversion, are force-dependent processes ( Fig. 4a ). See Supplementary Methods and Supplementary Fig. 11 for the detailed derivation of this model. 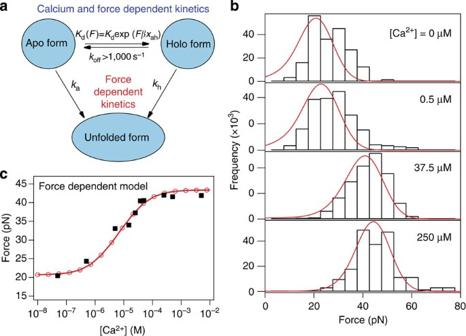Figure 4: A force-dependent binding model. (a) In this new kinetic model, both the unfolding kinetics of the calcium-free apo and the calcium-bound holo forms and their interconversion are force-dependent processes.xahis a parameter describing the dependency of dissociation constant on the applied force. We setkoff>1,000 s−1to reflect the fast interconversion between apo and holo forms. (b) The unfolding force histograms at various calcium concentrations (black bars) can be numerically fitted using theKdobtained from ITC and anxahof −0.7 nm based on the ‘force-dependent binding model’ (red lines). The negativexahindicates that force decreases the dissociation constant and makes the holo form more stable. Theχ2for the fittings to the histograms from top to bottom are 0.093, 0.059, 0.036 and 0.029, respectively. (c) This kinetic model can also describe the unfolding forces of G6 at different calcium concentrations. Red circles and black squares correspond to the numerically calculated data and the experimentally obtained data, respectively. Theχ2for the fitting is 0.22. Figure 4: A force-dependent binding model. ( a ) In this new kinetic model, both the unfolding kinetics of the calcium-free apo and the calcium-bound holo forms and their interconversion are force-dependent processes. x ah is a parameter describing the dependency of dissociation constant on the applied force. We set k off >1,000 s −1 to reflect the fast interconversion between apo and holo forms. ( b ) The unfolding force histograms at various calcium concentrations (black bars) can be numerically fitted using the K d obtained from ITC and an x ah of −0.7 nm based on the ‘force-dependent binding model’ (red lines). The negative x ah indicates that force decreases the dissociation constant and makes the holo form more stable. The χ 2 for the fittings to the histograms from top to bottom are 0.093, 0.059, 0.036 and 0.029, respectively. ( c ) This kinetic model can also describe the unfolding forces of G6 at different calcium concentrations. Red circles and black squares correspond to the numerically calculated data and the experimentally obtained data, respectively. The χ 2 for the fitting is 0.22. Full size image where K d and β are as defined above. K d (F) is the dissociation constant at a given force F , and x ah is the measure of the dependency of dissociation constant on the applied force. For x ah <0, force will decrease the dissociation constant and increase the binding affinity; for x ah >0, force will decrease the binding affinity; for x ah =0, force has no effect on the binding affinity. Here K d (F) is exponentially dependent on the applied force because force lowers the free energy barrier between the apo and holo forms linearly while K d (F) depends exponentially on the difference in free energy (see Supplementary Methods ). Similar to the force-independent binding model, to warrant a single unimodal unfolding force distribution for G6 at the intermediate calcium concentration, the k off should be higher than 1,000 s −1 in the force-dependent binding model ( Supplementary Fig. 12 ). Using this force-dependent binding model, the unfolding force histograms, at various [Ca 2+ ], can be fitted numerically using the K d obtained from ITC and a x ah of −0.7 nm ( Fig. 4b ). The negative x ah indicates that force decreases the dissociation constant and that the calcium-bound form is more stable under force. A stretching force of 10 pN increases the calcium-binding affinity of G6 by a factor of 5.5. Moreover, this model can also reproduce the average unfolding forces over the full range of calcium concentrations ( Fig. 4c ). Intriguingly, in this model, even at a stretching force of 20 pN (the unfolding force for calcium-free G6), the K d is actually much larger than the optimum K d used to ‘fit’ the experimental data using the force-independent model. This is due to the coupling of the interconversion of calcium-free and calcium-bound forms to their unfolding processes in the force-dependent binding model. It is worth mentioning that the force-dependent binding model more accurately predicts the slope of the force changes with respect to the [Ca 2+ ] than the force-independent model in combination with the artificially low K d . Therefore, these experimental data provide strong support for the force-dependent binding model. A further test of this model comes from measuring the pulling speed-dependent unfolding forces of G6 at the intermediate [Ca 2+ ] of 5 μM. The new force-dependent binding model satisfactorily predicts the experimentally obtained unfolding forces over the range of pulling speeds using the same parameters that were used to simulate the unfolding forces at various [Ca 2+ ]. In contrast, the force-independent binding model fails to reproduce the unfolding forces over the same range of pulling speeds ( Supplementary Fig. 13 ). We have also tested whether the experimental data can be fitted by other models, such as one that includes the presence of an additional force-revealed calcium-binding site in G6, and another that takes into account non-specific calcium binding to G6 ( Supplementary Fig. 14 ). Generally, the models that best reproduce the experimental data require an increase in overall calcium-binding affinity of G6 under force, regardless of the distinctive nature of the mechanism. The molecular origin of the force-enhanced calcium binding The detachment of the C-terminal latch helix of G6 from G2 has been proposed to be the key step of the activation of gelsolin upon calcium binding. In the crystal structure of activated gelsolin fragments, the C-terminal helix region is unstructured. We propose that force may facilitate the unfolding of the C-terminal extension to G6 and thus increase the calcium-binding affinity of G6. To test this hypothesis, we engineered a truncated version of G6 that lacks the last 19 residues of the C-terminal region ( Supplementary Fig. 15 ). This mutant, denoted G6_cut, mimics the rearrangement of the C-terminal helix by force. Unfortunately, because G6_cut is not as stable as G6, the polyprotein (GB1–G6_cut) 4 cannot be expressed in E. coli in a soluble form. Hence, we were not able to directly measure the calcium-binding affinity of G6_cut using single-molecule AFM. However, the monomer G6_cut protein can be expressed in E. coli with reasonable yield (5 mg per liter of Luria-Bertani medium). Thus, we measured the calcium-binding affinity of G6_cut using ITC. We found that G6_cut indeed showed an approximate sevenfold higher calcium-binding affinity when compared with full-length G6 in the absence of force. Such a binding affinity is equivalent to that of the full-length G6 under a stretching force of ~8 pN using single-molecule AFM. Since the C-terminal extension to G6 is close to the calcium-binding site of G6, it is probable that force could unfold this region and facilitate calcium binding. It is worth mentioning that even using the binding affinity for G6_cut, the unfolding forces of G6 at different [Ca 2+ ] still cannot be adequately ‘fitted’ by the force-independent binding model ( Supplementary Fig. 16 ). This further suggests that force-enhanced binding mechanism is important for the activation of gelsolin by calcium ions. Moreover, comparing the structures of apo and holo G6, the residues involved in calcium ion binding are distorted in the apo form ( Supplementary Fig. 1 ). During calcium activation of G6, the AB-strand pair moves together with the straightening of the long helix, which harbours one calcium-coordinating residue Glu692 (ref. 2 ). For calcium binding to induce a conformational change in the G6, the calcium-coordinating residues cannot, by definition, be in their optimal calcium-coordinating positions in the apo form. We suggest that putting force on the A-strand favors helix straightening and brings Glu692 closer to its optimal calcium-coordinating position. In future, detailed molecular dynamics simulations may help test such hypotheses as to the mechanisms underlying the force-enhanced calcium binding of G6. It is worth mentioning that the upper force limits needed to observe the force-enhanced calcium binding of G6 is the unfolding force of G6. If the force is >20 pN, it will trigger the unfolding of G6, leading to a decrease, instead of increase, of the calcium-binding affinity. Partial unfolding of a protein by force can sometimes be mimicked by increasing temperature or adding low concentrations of denaturants. We have measured calcium binding to G6 using ITC at an elevated temperature (37 °C), as well as in the presence of low concentrations of denaturants (0.8 M guanidinium chloride) ( Supplementary Fig. 17 ). However, the calcium-binding affinity decreased instead of increasing. This is probably because temperature and denaturant act on proteins globally, whereas force is a vector which can act on local structures within a protein. Therefore, they have different effects. We also have performed single-molecule AFM measurements of G6 in the absence and presence of calcium ions at pH 6 ( Fig. 5 ). The unfolding force for apo G6 increased slightly to ~23 pN at pH 6.0, indicating that G6 is mechanically somewhat more stable at low pH. However, the unfolding forces of G6 in the presence of micromolar to millimolar of calcium at pH 6.0 are obviously lower than those at pH 7.4. Although low pH may activate gelsolin, it decreases the calcium-binding affinity of G6. This indicates that the activation mechanism of G6 by low pH and calcium ions may be unique. 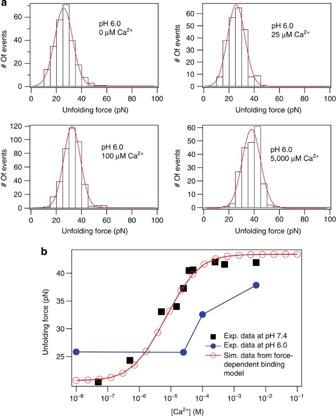Figure 5: The change of the unfolding forces for G6 at different [Ca2+] at pH 6. (a) The unfolding force histograms of G6 at different [Ca2+], pH 6 (pulling speed: 400 nm s−1). (b) The dependency of the unfolding forces of G6 on the concentrations of calcium ions at pH 7.4 and 6.0. Exp., experimental; Sim., Simulation. Figure 5: The change of the unfolding forces for G6 at different [Ca 2+ ] at pH 6. ( a ) The unfolding force histograms of G6 at different [Ca 2+ ], pH 6 (pulling speed: 400 nm s −1 ). ( b ) The dependency of the unfolding forces of G6 on the concentrations of calcium ions at pH 7.4 and 6.0. Exp., experimental; Sim., Simulation. Full size image Although it has been widely recognized that force can regulate ligand binding and Protein–protein interactions, the present finding that force can enhance the calcium ion binding affinity for G6 is, to our knowledge, the first experimental verification of this force-amplified ligand binding concept at the molecular level. Moreover, accurate measurement of the unfolding forces at different [Ca 2+ ] allowed us to quantitatively address the effect of force on the equilibrium binding constant. We found that a physiologically relevant force of ~10 pN could increase the binding affinity by more than fivefold. We propose a parameter, x ah , to quantify the dependence of the dissociation constant on the stretching force. The larger the absolute value of x ah , the greater is the effect of force on the binding affinity. A negative x ah indicates that the binding affinity is increased by force and a positive x ah reflects weaker binding under force. The kinetic model presented here can serve as a general physical model to deal with such complex force-dependent binding systems. However, this model may not be applicable for protein–ligand interactions that involve intermediate states in which the two-state binding assumption is not valid. Notably, the force-enhanced binding affinity demonstrated here is distinct from the well-established catch-bond mechanisms found in many ligand–receptor systems [38] , [39] , [40] . In the catch-bond mechanism, the lifetime of a bond increases with the applied force. However, lifetime is a kinetic quantity, while in our system the binding affinity is a thermodynamic quantity that describes the equilibrium characteristics of an interaction. Moreover, in our system, force is not directly applied between the ligand and receptor. Instead, regulation of the binding affinity is through the conformational change of a protein induced by an applied force. For rigid protein structures, the effect of force on the binding affinity may be not pronounced. However, for proteins with malleable structures, force could change the structures of both apo and holo states, leading to a change of binding affinity. Furthermore, the force-enhanced binding mechanism presented in this article is also conceptually different from the force-activated binding mechanism illustrated by others [10] , [11] , [12] , [13] . In our case, force only shifts the equilibrium between calcium-free and calcium-bound states. Even in the absence of force, a certain level of binding affinity is retained. In our experiments, we used the unfolding forces at different calcium concentrations as a probe for the force-dependent calcium binding by G6. This does not indicate that the force-enhanced calcium binding of G6 is due to the unfolding of G6. As shown in Supplementary Fig. 11 , force preferentially stabilizes the holo conformation over the apo conformation and thus increases the calcium-binding affinity of G6. The denatured G6 does not show any measurable calcium-binding affinity. Therefore, this leads to an upper boundary for the force-enhanced calcium-binding affinity. The maximum calcium-binding affinity of G6 is achieved at the unfolding force of holo G6. It is interesting to consider the physiological importance of stretching forces enhancing the binding affinity between calcium and G6. During the activation of gelsolin, calcium ion binding causes small conformational changes within the calcium-bound domains ( Fig. 1a,b , and Supplementary Fig. 1 ) and large conformational changes between domains [2] . It has been proposed that calcium binding to G6 controls the overall activation of gelsolin by releasing the tail latch that locks the inactive conformation of gelsolin [41] . This process may be required to create strain to dislodge the tail C-terminal helix, and ultimately, to reveal the actin-filament binding site on G2 ( Fig. 6 ). Thus, we propose that occupation of one or more calcium-binding sites within the first five domains of gelsolin will produce strain through the conformational restrictions placed on these domains by the tail C-terminal helix interaction with G2 ( Fig. 6a ), and as a consequence lead to a strain-induced increase in the binding of calcium to G6 ( Fig. 6b ). Consequently, gelsolin displays cooperativity in binding calcium ions that is mediated through changes in structure and, we propose, resultant changes in strain ( Fig. 6c ). We speculate that this produces a molecule that is finely tuned to react to [Ca 2+ ] changes and at the same time contains a safety switch at inappropriate calcium levels. Further structure biology and molecular dynamics simulations studies will be needed to characterize intermediate activation conformations to verify the proposed role of strain in the activation process. 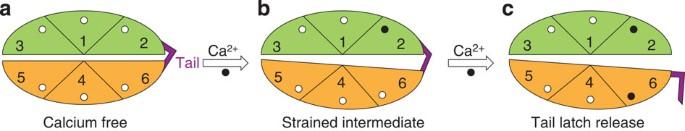Figure 6: Cartoon highlighting the initial activation stages of gelsolin. (a) Six-domain gelsolin contains a homologous calcium-binding site in each domain (white circles) and a C-terminal tail that interacts with domain 2 to lock the inactive conformation (coloured in purple). (b) Occupation of any of these sites by a calcium ion will begin the activation process that drives conformational reorganization and concomitantly creates inter-domain strain, leading to the C-terminal tail under tension. Here we show a calcium ion occupying the site on G2. Greater strain may be induced through filling more of the calcium-binding sites. (c) The resulting inter-domain strain will increase the affinity of G6 for calcium, resulting in calcium ion binding to G6 and the release of the tail latch, which in turn exposes the F-actin-binding site on G2. Figure 6: Cartoon highlighting the initial activation stages of gelsolin. ( a ) Six-domain gelsolin contains a homologous calcium-binding site in each domain (white circles) and a C-terminal tail that interacts with domain 2 to lock the inactive conformation (coloured in purple). ( b ) Occupation of any of these sites by a calcium ion will begin the activation process that drives conformational reorganization and concomitantly creates inter-domain strain, leading to the C-terminal tail under tension. Here we show a calcium ion occupying the site on G2. Greater strain may be induced through filling more of the calcium-binding sites. ( c ) The resulting inter-domain strain will increase the affinity of G6 for calcium, resulting in calcium ion binding to G6 and the release of the tail latch, which in turn exposes the F-actin-binding site on G2. Full size image A second area where strain-induced calcium binding may be important is in gelsolin’s interactions with actin. Based on crystal structures, the linker regions connecting G1–G2 and G3–G4 of gelsolin are very much elongated when it is bound to the actin filament [2] . The elongation of a peptide chain typically requires a tensile force. Based on simple polymer elasticity models, such as the WLC model or the freely-jointed chain model, activated gelsolin typically will be subjected to a tensile force of several piconewtons (see Supplementary Methods for detailed calculation). Such minute forces are sufficiently large to alter the calcium-binding affinity to gelsolin and thus its threshold for calcium activation mechanism. Furthermore, gelsolin undoubtedly undergoes changes in tension as it wraps itself over the surface of the actin filament during the severing process. Fluctuations in the filament will also create strain since gelsolin interacts with three actin protomers and encircles the filament. Should the force-enhanced calcium ion binding be common to the other domains of gelsolin (G1–G5), then this suggests that calcium binding will favour the portion of gelsolin that is bound to a filament over the free gelsolin pool. Thus, we speculate that at close to threshold calcium levels, gelsolin will remain bound to the filament and severing will be driven to completion, while free gelsolin may be able to return to the quiescent state through calcium dissociation. Quantifying the tensile force in gelsolin and other proteins under physiological conditions is challenging due to the lack of efficient in vivo force sensors. Nevertheless, a common trend is emerging that several proteins that regulate the force-generating actin polymerization machine are themselves subjected to force regulation. We are left with the question as to whether the force-dependent change in calcium-binding affinity is unique to G6 or a common feature shared by all gelsolin domains. Addressing this question will be an important step towards further understanding the activation mechanism of gelsolin. Due to the similar sizes of all gelsolin domains, it is not possible to assign different unfolding peaks for individual domains, within full-length gelsolin, to probe their calcium-binding affinities. Other techniques, such as using forster resonance energy transfer pairs to label the two ends of the G6 domain within full-length gelsolin may allow simultaneous measurement of the fluorescence change upon stretching in single-molecule AFM studies, and thus might open up the opportunity to study G6 within full-length gelsolin in the future. Protein engineering The gene encoding (GB1–G6) 4 hybrid polyprotein was constructed using standard molecular biology techniques to splice GB1 and G6 (P06396) in an iterative approach. (GB1–G6) 4 was expressed in BL21 and purified by Ni 2+ -affinity chromatography. EGTA (1 mM) was added to the protein sample to remove the residual free Ca 2+ in buffer. Then the purified polyprotein sample was dialyzed and kept at 4 °C in Tris-HCl buffer (10 mM, pH 7.4, 10 mM NaCl) at a concentration of 0.3 mg ml −1 . Single-molecule AFM Single-molecule AFM experiments were carried out on a commercial AFM (ForceRobot 300, JPK, Berlin, Germany). All the force-extension experiments were carried out in Tris-HCl buffer (10 mM, pH 7.4, 10 mM NaCl and 0–5 mM CaCl 2 calibrated with EGTA [42] ). Protein sample (150 μl) was directly deposited on a freshly cleaved glass surface for 20 min. Then, the sample chamber was filled with 1.5 ml buffer before the measurement. Typically, experiments proceeded <12 h to avoid the concentration changes in Ca 2+ from evaporation of water. The spring constant of the AFM cantilevers (Biolever-RC-150VB-70 from Olympus) was calibrated using the equipartition theorem before each experiment, with a typical value of 6 pN nm −1 , and was recalibrated every 4–6 h during each experiment. The pulling speed was 400 nm s −1 for all traces unless otherwise indicated. How to cite this article: Lv, C. et al. Single-molecule force spectroscopy reveals force-enhanced binding of calcium ions by gelsolin. Nat. Commun. 5:4623 doi: 10.1038/ncomms5623 (2014).